Intestinal-derived FGF15 protects against deleterious effects of vertical sleeve gastrectomy in mice Bariatric surgeries such as the Vertical Sleeve Gastrectomy (VSG) are invasive but provide the most effective improvements in obesity and Type 2 diabetes. We hypothesized a potential role for the gut hormone Fibroblast-Growth Factor 15/19 which is increased after VSG and pharmacologically can improve energy homeostasis and glucose handling. We generated intestinal-specific FGF15 knockout (FGF15 INT-KO ) mice which were maintained on high-fat diet. FGF15 INT-KO mice lost more weight after VSG as a result of increased lean tissue loss. FGF15 INT-KO mice also lost more bone density and bone marrow adipose tissue after VSG. The effect of VSG to improve glucose tolerance was also absent in FGF15 INT-KO . VSG resulted in increased plasma bile acid levels but were considerably higher in VSG-FGF15 INT-KO mice. These data point to an important role after VSG for intestinal FGF15 to protect the organism from deleterious effects of VSG potentially by limiting the increase in circulating bile acids. Obesity has become a growing epidemic, where associated complications such as cardiovascular morbidity, Type 2 diabetes, and insulin resistance pose major health care challenges [1] . Current pharmacological treatments for obesity include <10 FDA-approved drugs, all of which demonstrate modest effect sizes [2] . Although invasive, bariatric surgery is the most effective treatment for sustained weight loss and also improves glycemic control better than conventional weight-loss therapies [3] , [4] , [5] . The gastrointestinal tract plays an important role in regulating many of the potent metabolic effects of bariatric surgery leading to reduced body weight and improved glucose metabolism. An important weight-independent effect of bariatric surgery is the alteration of enterohepatic bile acid circulation resulting in increased plasma bile levels as well as altered bile acid composition in rodents [6] , [7] and humans [8] , [9] . We and others have hypothesized that changes in the enterohepatic metabolism play important role in the potent metabolic effects of vertical sleeve gastrectomy (VSG) and Roux-Y Gastric Bypass (RYGB) [10] , [11] . We identified bile acid signaling through the nuclear ligand-activated farnesoid X receptor (FXR) as a potential link for mediating the beneficial effects of elevated bile acids following bariatric surgery. We also reported that bile acids are increased after VSG and that FXR is essential for the positive effects of bariatric surgery on weight loss and glycemic control [6] , [12] . Unlike wild-type mice, FXR−/− mice do not maintain body weight loss and do not have improved glucose tolerance after VSG or after bile diversion to the ileum [12] , [13] . These studies highlighted the importance of enterohepatic circulation in the metabolic effects following bariatric surgery. Absorbed bile acids activate intestinal FXR and its downstream target FGF15/19 (mouse/human ortholog, respectively). FGF15/19 is a gut hormone expressed in ileal enterocytes of the small intestine and is released postprandially in response to bile acid absorption among other stimuli [14] , [15] , [16] , [17] . Once released from the ileum, FGF15/19 enters the portal venous circulation and travels to the liver where FGF15/19 binds to its receptor FGFR4 and represses de novo bile acid synthesis and gallbladder filling [14] . Pharmacological administration of FGF15/19 has potent effects to reduce bile acid levels and secretion at the level of both the liver and the gallbladder [18] , [19] . Importantly, pharmacological administration of FGF19 reduces body weight and improves glucose regulation in rodents [20] . FGF15/19 stimulates protein and glycogen synthesis, while reducing gluconeogenesis, hepatic triglycerides, and cholesterol [18] , [19] . FGF19 levels also rise 2–4 h postprandially, which is considerably later than insulin and GLP-1 [17] . These notable metabolic actions and protein engineering has made FGF19 analogues attractive candidates for the treatment of type 2 diabetes and hepatic lipid disorders with a number of clinical trials under way [10] , [21] , [22] , [23] . Pharmacologically elevating FGF15/19 levels in rodent models of metabolic disease results in multiple metabolic benefits including increased energy expenditure, reduced adiposity, and improved lipid and glucose homeostasis [24] , [25] , [26] , [27] , [28] . FGF19 levels are lower in patients with obesity, without a strong association to glucose metabolism nor insulin sensitivity [29] , [30] , [31] , [32] , [33] . However, other studies report that basal FGF19 levels are inversely correlated to glucose metabolism or insulin sensitivity [34] , [35] and nonalcoholic fatty liver disease (NAFLD) [36] , [37] . Most importantly, fasting and postprandial plasma FGF19 levels in humans [22] , [32] , [33] , [38] , [39] , [40] and ileal FGF15 expression in mice (as shown in the present studies) increase after VSG. These data point to FGF15/19 as a potential target to mediate VSG’s effects to produce sustained weight loss and improved glucose tolerance. To test the hypothesis of whether FGF15 plays a role in the metabolic improvements after bariatric surgery, we generated a novel mouse model of intestinal-specific FGF15 knock out (VilCreERT2; Fgf15 f/f ) and controls, which were maintained on a 60% high-fat diet (HFD) before and after undergoing Sham or VSG surgery. Here we report that intestinal-derived FGF15 is necessary to prevent excessive bile acid increases and prevent the consequent loss in muscle and bone mass, the improvement in peripheral blood glucose regulation, and the decrease in hepatic cholesterol after VSG. These findings point to an important role for FGF15 in the regulation of multiple metabolic parameters following VSG. Intestinal FGF15 expression increases and prevents muscle mass loss after VSG in mice Numerous reports have also shown that plasma FGF19 levels increase after weight-loss surgeries [22] , [32] , [33] , [38] , [39] , [40] . Due to the lack of commercially available and validated FGF15 assays, we were unable to measure circulating FGF15 levels after VSG in mice [41] , [42] . However, our data show that ileal FGF15 expression increases after VSG in mice (Fig. 1a ). These data point to FGF15/19 as a potential target to mediate the effects of weight-loss surgery. Fig. 1: Intestinal FGF15 expression increases and prevents muscle mass loss after VSG in mice. a FGF15 RNA expression in duodenum, jejunum and ileum in control Sham and VSG mice fed 60% HFD. Intestinal mucosa was collected 15 min post mixed meal gavage ( n = 6 Sham and 7 VSG). b Experimental timeline. c Body weight and d food intake before surgery. e Body weight after surgery. f Fat body mass and g lean body mass before and after surgery. h Cumulative food intake and i energy efficiency for weeks 1–8 after surgery. j Food intake, k fecal energy and l absorbed energy during week 11 after surgery. Animal number: Control Sham ( n = 6), Control VSG ( n = 8), FGF15 INT-KO Sham ( n = 8), FGF15 INT-KO VSG ( n = 5). Data are shown as means ± SEM. Panels a , c , and d were analyzed with Student’s two-tailed t test. Panels e – l were analyzed with two-way ANOVA with Tukey’s post hoc test. * p < 0.05. Full size image Global ablation of FGF15 in FGF15−/− mice resulted in impaired glucose tolerance [18] , [19] , but in our hands, these mice are surprisingly protected against diet-induced obesity [43] .FGF15 is highly expressed in the developing mouse brain [44] , [45] , [46] . Expression of FGF15 in the adult mouse becomes limited to the distal intestine and dorsal medial hypothalamus [14] , [15] , [47] . Thus, we speculate that the total body knockouts have impaired development of the CNS, which likely contributes to their reduced weight gain on a HFD. These issues make it difficult to use the total body knockout to determine critical aspects of FGF15 function in adult animals. Therefore, we generated a FGF15 flox/flox mouse to test specific hypotheses about the tissue-specific role of FGF15 in metabolism after VSG. The FGF15 flox/flox mice were built using CRISPR-Cas9 with LoxP sites flanking exon 2 of the FGF15 gene. We bred these mice to VilCreERT2 mice and administered tamoxifen (intraperitoneal, 3 doses/150 mg/kg; Fig. 1b ) to FGF15 INT-KO (VilCreERT2; FGF15 flox/flox) and Controls (6 VilCreERT2, 4 FGF15 flox/flox, and 4 FGF15 flox/+ were combined as there were no differences in the phenotypes of these animals; Fig. 1b ). After the studies were completed, we validated exon 2 excision within ileal mucosa (where FGF15 is most highly expressed) in all mice (Supplementary Fig. 1 ). FGF15 INT-KO Sham and VSG mice had undetectable expression of ileal FGF15 , with no significant alterations in ileal FXR expression, although there was a trend of decreased expression in FGF15 INT-KO Sham compared to Control Sham (Supplementary Fig. 1a, b ). All mice received tamoxifen at the same time, and a week later were placed on 60% high-fat diet (HFD; Fig. 1a ). Prior to surgery, Control and FGF15 INT-KO mice had similar body weight increase in response to HFD, without differences in food intake, fat and lean mass (Fig. 1c, d, f, g ). After 8 weeks of being on HFD, each mouse underwent either a Sham or VSG procedure and was returned to HFD four days after surgery. VSG removes ~80% of the stomach along the stomach curvature (Fig. 1a ). As expected, Control mice receiving VSG had sustained weight loss compared to Control Sham mice, and that weight loss came mostly from loss of fat mass (Fig. 1e, f ). Control VSG mice maintained their lean mass even after surgery, as we have shown before [48] . FGF15 INT-KO VSG mice also lost a significant amount of weight, but 9 weeks post-surgery their body weight was significantly lower compared to Control VSG (Fig. 1e ). Although FGF15 INT-KO VSG mice lost fat mass, surprisingly they also lost a significant amount of lean mass and this loss was significantly greater than when compared to Control VSG and both Sham groups (Fig. 1f, g ). Cumulative food intake and the average energy efficiency (change in body weight divided by food intake) for the 8 weeks after surgery showed that the body weight loss observed in FGF15 INT-KO VSG mice was not a result of decreased food intake (Fig. 1h, i ). This introduced the possibility that the loss of intestinal FGF15 leads to increased malabsorption following VSG. We measured the absorbed energy by bomb calorimetry 11 weeks after surgery. The average daily food intake was not different between the groups (Fig. 1j ). However, the fecal energy output was reduced in FGF15 INT-KO VSG mice compared to Control VSG and FGF15 INT-KO Sham mice (Fig. 1k ). Given that all mice were on the same diet, FGF15 INT-KO VSG mice had increased their absorption of calories from ingested food (Fig. 1l ). Thus, the additional weight and lean mass loss in FGF15 INT-KO VSG was not secondary to nutrient malabsorption. Loss in muscle mass is accompanied by decreased strength and skeletal muscle fiber size in FGF15 INT-KO VSG mice Previous data has shown that exogenous administration or genetic overexpression of FGF19 decreases body weight and adiposity [20] , [24] , [25] , [26] , [27] , [28] , but prevents muscle mass wasting by enlarging muscle fiber size and protecting muscle from atrophy [49] . In addition to significant loss of muscle mass in FGF15 INT-KO VSG mice (Fig. 1g ), we observed a trend of decreased grip strength (9 weeks post-surgery) and soleus muscle fiber size in these mice (Supplementary Fig. 2a, b ). Moreover, a distribution analysis of the fiber size showed that FGF15 INT-KO VSG mice have a rightward shift towards an increased number of smaller and a lower number of larger soleus fibers (Supplementary Fig. 2c ). To further examine the atrophy-related pathways in soleus muscle, we measured circulating Myostatin (GDF8) and Activin A levels and the soleus muscle expression of their downstream targets, muscle-specific E3 ubiquitin ligases Atrogin 1 and MuRF1. We did not observe any differences in the plasma Myostatin and Activin A levels, nor the RNA expression of Atrogin 1 (encoded by Fbxo32 ) and MuRF1 (encoded by Trim63 ) in soleus muscle (Supplementary Fig. 2d–g ). Next, we examined plasma levels of IGF1 and FGF21 as anti and pro-atrophy mediators in skeletal muscle. Twelve weeks after surgery postprandial plasma levels of IGF1 were decreased in FGF15 INT-KO VSG mice compared to Control VSG (Supplementary Fig. 2h ). Studies have indicated that FGF21 levels increase with fasting and FGF21 is necessary for the fasting-induced muscle mass and force loss [50] . FGF15 INT-KO VSG mice had increased plasma levels of FGF21 compared to Control VSG and FGF15 INT-KO Sham mice (Supplementary Fig. 2i ). In addition, there was a significant negative correlation between muscle mass and plasma FGF21 levels (Supplementary Fig. 2j ). Circulating amino acid levels 6-weeks post-surgery were not different among the groups (Supplementary Fig. 2k ). FGF15 INT-KO VSG mice did not show differences in small bowel biometry (Supplementary Fig. 3a–c ). The large bowel weight was significantly less in FGF15 INT-KO VSG compared to FGF15 INT-KO Sham mice (Supplementary Fig. 3d ). However, there was also a trend toward decreased large bowel weight in Control VSG compared to Control Sham mice, suggesting that decrease in large bowel weight could be related to decreased body weight of the VSG groups (Supplementary Fig. 3d ) [51] . The ratio of large bowel weight/length was significantly reduced in both VSG groups compared to Control Sham but was not significantly different compared to FGF15 INT-KO Sham mice (Supplementary Fig. 3f ). Further analysis of ileum cross-sections showed no differences in villi height, crypt depth or the ratio of villi height/crypt depth (Supplementary Fig. 3g–i ). Intestinal-derived FGF15 partially preserves bone and bone marrow adipose tissue (BMAT) loss following VSG Previous studies in our lab have shown that loss of bone and BMAT following VSG is independent of body weight and diet [52] . In the current study, VSG caused a precipitous loss of trabecular and cortical bone loss in FGF15 INT-KO mice. Specifically, FGF15 INT-KO VSG mice had decreased trabecular bone volume fraction (Tb. BV/TV), trabecular bone mineral density (Tb. BMD), and trabecular connective density (Conn. Dens) (Fig. 2a–d ). Although the thickness of the trabecular bone (Tb. Th) was not altered, the trabecular number (Tb. N) was decreased, while the spacing between trabeculae was increased (Tb. Sp) in FGF15 INT-KO VSG mice (Fig. 2e–g ). Cortical thickness (Ct. Th), bone area (Ct. BA/TA), and bone mineral density (Ct. BMD) were reduced by VSG and further decreased by lack of intestinal-derived FGF15 (Fig. 2h–k ). Fig. 2: Intestinal-derived FGF15 partially preserves bone and bone marrow adipose tissue (BMAT) loss following VSG. a 3D images of trabecular bone, scale bars 500 μm. b Trabecular bone volume fraction (Tb. BV/TV), c trabecular bone mineral density (Tb. BMD), d trabecular bone connective density (Conn. Des) and e trabecular number (Tb. N), f thickness of the trabecular bone (Tb. Th), g spacing between trabeculae (Tb. Sp). h 3D images of mid-cortical bone, scale bars 500 μm. i Thickness of the cortical bone (Ct. Th). j Cortical bone area (Ct. BA/TA) and k cortical bone mineral density (Ct. BMD). l Tibial BMAT was visualized by osmium staining. m , n Representative sections from proximal and distal tibiae were stained with H&E and are shown at ×100 magnification, scale bars 200 μm. l Tibial BMAT was quantified relative to total bone volume after osmium staining within the indicated regions as shown in ( o ) proximal Tibia ( ① - ② ), p growth plate (G/P) to tibia/fibula junction (T/F J) ( ① - ③ ), q distal tibia is T/F J to distal end ( ③ - ④ ). Animal number: Control Sham ( n = 5), Control VSG ( n = 8), FGF15 INT-KO Sham ( n = 7), FGF15 INT-KO VSG ( n = 5). Data are shown as means ± SEM. * p < 0.05 (two-way ANOVA with Tukey’s post hoc test). Full size image Consistent with our previous studies, both “regulated” bone marrow adipose tissue, BMAT (rBMAT) in proximal tibia and “constitutive” BMAT (cBMAT) in distal tibia were decreased by VSG (representative images Fig. 2m, n ) [52] , [53] . Interestingly, loss of intestinal FGF15 caused a baseline reduction of rBMAT in proximal tibia ranging from growth plate (GP) to tibia/fibula junction (T/F J), with nearly complete depletion after VSG (Fig. 2m, o, p ). Although the distal tibial cBMAT of Sham mice was unaffected by loss of intestinal FGF15, this BMAT depot was more thoroughly depleted in FGF15 INT-KO VSG mice compared to Control VSG mice (Fig. 2n, q ). Loss of intestinal FGF15 increases circulating fibroblast growth factor 23 (FGF23) and erythropoietin (EPO) levels after VSG Fibroblast growth factor 23 (FGF23), the third member of the endocrine FGFs in addition to FGF15/19 and FGF21, is a bone-derived hormone that regulates mineral homeostasis and consequently bone mineral density [54] . Plasma FGF23 levels were elevated almost 20,000-fold in FGF15 INT-KO VSG mice (Fig. 3a ). Plasma phosphate and 25 (OH) vitamin D levels were unaffected (Fig. 3b, c ). To investigate the cause for increased plasma FGF23 levels, we measured circulating erythropoietin (EPO), a known regulator of FGF23 and bone loss [55] , [56] . EPO was also increased by 15,000-fold in FGF15 INT-KO VSG mice (Fig. 3d ). Increased plasma FGF23 and EPO levels are often observed in anemia. Hemoglobin levels were decreased in FGF15 INT-KO VSG compared to FGF15 INT-KO Sham mice (Fig. 3e ). Plasma ferritin levels were unaffected (Fig. 3f ). Consistent with high levels of EPO, heart to body weight ratio (Fig. 3g ) was increased in FGF15 INT-KO VSG mice. Moreover, H&E stains in liver sections showed zonal injury pattern (Fig. 3h ). Zone 3 around the central hepatic veins appeared paler compared to zones 1 and 2 (Fig. 3h ). These patterns are consistent with relative hypoxia, possibly secondary to anemia. The expression of hypoxia-inducible factor 2 alpha ( Hif2α ) and its target genes were upregulated in the duodenum following VSG and independent of genotype, specifically those genes transcribing the iron transporters divalent metal transporter Dmt1 (encoded by Slc11a2 ), duodenal cytochrome B Dcytb (encoded by Cybrd1 ), and Ferroportin (encoded by Slc401a1 ) (Fig. 3i ). Duodenal expression of hepcidin ( Hamp ) was not altered by VSG or lack of gut-derived FGF15 expression (Fig. 3i ). Lastly, iron content in cecal contents was not different between the groups but showed a trend of increased levels in both VSG groups (Fig. 3j ). Fig. 3: Loss of intestinal FGF15 increases circulating fibroblast growth factor 23 (FGF23) and erythropoietin (EPO) levels after VSG. Plasma levels of a FGF23, b phosphate, c 25(OH) vitamin D, d erythropoietin, e hemoglobin and f ferritin. g Heart to body weight ratio. h H&E stain of liver sections, CV = central vein, PV = portal vein, Zones 1–3, scale bars 100 μm. i RNA expression of Dmt1, Dcytb , Hamp , Slc401a1 (Fpn) and Hif2α in duodenum. j Iron levels in cecal contents. Animal number for ( a – f ) and ( i , j ): Control Sham ( n = 5), Control VSG (n = 8), FGF15 INT-KO Sham ( n = 8), FGF15 INT-KO VSG ( n = 5). Animal number for g: Control Sham ( n = 6), Control VSG ( n = 8), FGF15 INT-KO Sham (n = 8), FGF15 INT-KO VSG ( n = 5). Data are shown as means ± SEM. * p < 0.05 (two-way ANOVA with Tukey’s post hoc test). Full size image Loss of intestinal FGF15 increases circulating total GLP-1 levels and increases gastric emptying after VSG Four-hour fasted blood glucose concentrations were not different among any of the four groups, but insulin concentrations and HOMA-IR were lower in FGF15 INT-KO VSG compared to FGF15 INT-KO Sham (Fig. 4a–c ). As expected, we saw improvements in glucose tolerance in Control VSG compared to Control Sham mice six- and nine-weeks post-surgery (Fig. 4d, e ). To our surprise, there was no difference in glucose tolerance between FGF15 INT-KO VSG and FGF15 INT-KO Sham mice (Fig. 4d, e ). Fig. 4: FGF15 INT-KO mice remain glucose intolerant despite significant body weight loss after VSG. a Fasting (4 h) blood glucose, b fasting (4 h) insulin levels and c HOMA-IR after surgery. d Intraperitoneal glucose tolerance test (ipGTT; 2 g/kg) performed 6-weeks post-surgery and Area Under the Curve (AUC). e Intraperitoneal glucose tolerance test (ipGTT; 2 g/kg) performed 9 weeks post-surgery and Area Under the Curve (AUC). f Mixed meal tolerance test (MMTT) performed 10 weeks post-surgery. g Gastric emptying rate measured by acetaminophen levels at 15 min post mixed meal. h Insulin levels at baseline (4 h fast) and 15 min post mixed meal. i Total GLP-1 levels at baseline (4 h fast) and 15 min post mixed meal. Animal number ( a – f ) and ( h , i ): Control Sham ( n = 6), Control VSG ( n = 8), FGF15 INT-KO Sham ( n = 8), FGF15 INT-KO VSG ( n = 5). Animal number g: Control Sham ( n = 6), Control VSG ( n = 7), FGF15 INT-KO Sham ( n = 8), FGF15 INT-KO VSG ( n = 5). Data are shown as means ± SEM. * p < 0.05 (two-way ANOVA with Tukey’s post hoc test). Full size image Next, we challenged mice with a mixed meal for the assessment of postprandial glucose excursion, insulin, and GLP-1 response. Acetaminophen, which is rapidly absorbed once it leaves the stomach was added to the mixed meal to assess gastric emptying rate. FGF15 INT-KO Sham mice had a similar glucose excursion curve, but decreased gastric emptying rate compared to Control Sham mice (Fig. 4f, g ). Both VSG groups responded to the mixed meal with similar glucose excursion curves (Fig. 4f ), significantly higher than their Sham controls as a result of increased gastric emptying rate (Fig. 4g ). Despite similar glucose excursion, FGF15 INT-KO VSG mice showed significantly higher gastric emptying rate (indicated by the greater plasma acetaminophen levels) compared to Control VSG mice (Fig. 4g ). Basal and postprandial insulin levels were increased in both VSG groups compared to Sham controls (Fig. 4h ). Interestingly, basal and postprandial total GLP-1 levels were significantly higher in FGF15 INT-KO VSG mice compared to all other groups (Fig. 4i ). Loss of intestinal FGF15 results in aberrant hepatic lipid and glycogen metabolism following VSG FGF15 INT-KO VSG had increased liver to body weight ratio (Fig. 5a ). Assessment of glycogen stores revealed that FGF15 INT-KO VSG have decreased liver glycogen and a trend toward higher skeletal muscle (tibialis anterior) glycogen content (Supplementary Fig. 4a, b ). Postprandial plasma alanine aminotransferase (ALT) levels, a predictor of liver injury, and plasma cholesterol levels trended to be reduced in both VSG groups compared to Sham controls (Fig. 5b, c ), without changes in plasma-free fatty acids or plasma triglycerides (Fig. 5d, e ). Fig. 5: Loss of intestinal FGF15 results in aberrant hepatic lipid metabolism following VSG. a Liver weight normalized to body weight. b Alanine aminotransferase (ALT) plasma levels. c Plasma cholesterol. d Plasma-free fatty acids (FFA) and e Plasma triglycerides (postprandial, 12 weeks post-surgery). f Total hepatic cholesterol. g Hepatic esterified cholesterol. h Hepatic triglycerides. i Hepatic free fatty acids. Hepatic RNA expression of cholesterol synthesis gene j . Hmcgr and cholesterol export genes k . Abcg5 and l . Abcg8 . Animal number for ( a – i ) and ( k , l ): Control Sham ( n = 5), Control VSG ( n = 8), FGF15 INT-KO Sham ( n = 8), FGF15 INT-KO VSG ( n = 5). Animal number for j: Control Sham ( n = 5), Control VSG ( n = 8), FGF15 INT-KO Sham ( n = 7), FGF15 INT-KO VSG ( n = 5). Data are shown as means ± SEM. * p < 0.05 (two-way ANOVA with Tukey’s post hoc test). Full size image Analysis of hepatic lipids revealed an increased cholesterol and esterified cholesterol levels in FGF15 INT-KO VSG mice (Fig. 5f, g ). Hepatic triacylglycerols were decreased in Control VSG compared to Control Sham mice, but remained at similar levels between FGF15 INT-KO Sham and FGF15 INT-KO VSG mice (Fig. 5h ). There was a trend toward decreased hepatic free fatty acids in both VSG groups compared to Sham controls (Fig. 5i ). Surprisingly, the cholesterol synthesis rate-limiting gene, 3-hydroxy-3-methyl-glutaryl-glutaryl-coenzyme A reductase, Hmg-CoA reductase ( Hmcgr ), was upregulated in FGF15 INT-KO Sham compared to Control Sham mice, but reduced after VSG in FGF15 INT-KO VSG mice (Fig. 5j ). Next, we measured the expression in hepatic cholesterol efflux pump-ATP-binding cassette, sub-family G, members 5 and 8 ( Abcg5 and Abcg8 ) and found that their expression was decreased in FGF15 INT-KO VSG mice (Fig. 5k, l ). These data suggest that despite decreased cholesterol synthesis, there is attenuated cholesterol export leading to elevated liver cholesterol content in FGF15 INT-KO VSG mice. The hepatic expression of FXR was similar in Control and FGF15 INT-KO mice (Supplementary Fig. 5a ). We did see a trend of decreased expression of FXR in both VSG groups compared to their respective Sham groups (Supplementary Fig. 5a ). FXR target small heterodimer partner, SHP , was not significantly different, but showed a trend for decreased expression in both VSG groups. (Supplementary Fig. 5b ). Fatty acid oxidation and lipid metabolism genes fatty acid synthase ( FAS ) and peroxisome proliferator-activated receptor alpha (PPAR alpha) were decreased in FGF15 INT-KO VSG mice compared to FGF15 INT-KO Sham controls (Supplementary Fig. 5c, d ). Although not significant, there was a trend of decreased expression of these genes in Control VSG compared to Control Sham mice (Supplementary Fig. 5c, d ). PPAR alpha target gene, Carnitine palmitoyltransferase 1A ( Cpt1a ) essential for converting long-chain fatty acids into energy (lipogenesis), showed a trend toward decreased expression after VSG in FGF15 INT-KO but not Control mice (Supplementary Fig. 5e ). Interestingly, cluster of differentiation 36 ( CD36 ), a cell surface protein that imports fatty acids, was increased in FGF15 INT-KO VSG compared to Control VSG mice (Supplementary Fig. 5f ). Intestinal FGF15 regulates enterohepatic bile acid metabolism following VSG FGF15 is expressed in ileal enterocytes of the small intestine and released postprandially in response to bile acid absorption. Consistent with this role to inhibit bile acid production, plasma and cecal content concentrations of bile acids are higher in mice lacking intestinal FGF15 (Fig. 6a, b ). Moreover, plasma bile acid composition revealed higher levels of TCA (taurocholate), CDCA (chenodeoxycholate), DCA (Deoxycholate), TDCA (taurodeoxycholate), and TCDCA (Fig. 6d ). VSG has been shown to alter both the concentration and composition of bile acids. Therefore, we assessed the role that FGF15 might play in the effect of VSG to alter bile acids. Control VSG mice had a trend of increased plasma bile acid levels, with higher levels of TαMCA (tauro-α-muricholate)/ TβMCA (tauro-β-muricholate), TCA, DCA, and TDCA levels (Fig. 6d , Supplementary Fig. 6 ). FGF15 INT-KO VSG mice had much higher plasma bile acid levels, but normal cecum content of bile acid levels when compared to Control VSG and FGF15 INT-KO Sham mice (Fig. 6a, b ). FGF15 INT-KO VSG mice also had higher plasma TαMCA/TβMCA levels (similar to Control VSG), but also high levels of TCA, CDCA, DCA, TDCA, CA (cholate) (Fig. 6D , Supplementary Fig. 6 ). The levels of hydrophobic bile acids (GCA/glycocholate, CA/cholate, CDCA/chenodeoxycholate, DCA/deoxycholate, LCA/lithocholic acid) in plasma were increased by more than two-fold in FGF15 INT-KO VSG compared to Control VSG mice (Fig. 6e , Supplementary Fig. 6 ). Hepatic total bile acid levels were not different but showed a trend of decreased levels in both VSG groups (Fig. 6c ). The ratios of cholesterol to bile acids in plasma, liver, and cecal content showed that lack of gut-derived FGF15 after VSG drives a system for increased bile acids in plasma and increased cholesterol in the liver (Supplementary Fig. 7a–c ). Not surprisingly, lack of intestinal FGF15 resulted in higher expression of the bile acid synthesis gene Cyp7a1 in FGF15 INT-KO Sham compared to Control Sham mice (Fig. 6f ). However, despite the fact that FGF15 INT-KO VSG mice lack intestinal FGF15 and have increased plasma bile acid levels, their expression of hepatic bile acid synthesis genes cholesterol 7a-hydroxylase (Cyp7a1) , sterol 12-alpha-hydroxylase (Cyp8b1), and sterol 27-hydroxylase (Cyp27a1) were decreased (Fig. 6f–h ). Fig. 6: Intestinal FGF15 regulates enterohepatic bile acid metabolism following VSG. a Total plasma bile acid levels. b Cecal contents total bile acid levels. c . Hepatic total bile acids. d Plasma bile acid composition. e Hydrophobic plasma bile acid levels. Hepatic RNA expression of bile acid synthesis genes. f Cyp7a1 , g Cyp8b1 and h Cyp27a1 . Hepatic RNA expression of bile acid uptake genes i Slc10a1 (coding for Ntcp) and j Oatp4 . k Ileum RNA expression of bile acid uptake gene Slc10a2 (coding for Asbt). Animal number for ( b ), ( c ), ( f – j ): Control Sham ( n = 5), Control VSG ( n = 8), FGF15 INT-KO Sham ( n = 8), FGF15 INT-KO VSG ( n = 5). Animal number for ( a ), ( d ), ( e ): Control Sham ( n = 5), Control VSG ( n = 7), FGF15 INT-KO Sham ( n = 6), FGF15 INT-KO VSG ( n = 5). Animal number for k: Control Sham (n = 5), Control VSG ( n = 7), FGF15 INT-KO Sham ( n = 8), FGF15 INT-KO VSG ( n = 5). Data are shown as means ± SEM. * p < 0.05 (two-way ANOVA with Tukey’s post hoc test). Full size image Next, we measured the expression of hepatic and ileal bile acid uptake transporters. The expression of Slc10a1 (coding for liver bile acid transporter Ntcp) and Oatp4 was decreased in FGF15 INT-KO VSG mice (Fig. 6i, j ). We did not see differences in the expression of bile acid transporter Slc10a2 (coding for apical sodium-dependent bile acid transporter, Asbt) in the ileum (Fig. 6k ). These data suggest that bile acid uptake by liver is reduced in FGF15 INT-KO VSG mice, potentially contributing to the increased plasma bile acid levels. Intestinal FGF15 modulates microbiota in cecal content Changes in gut microbiota composition are considered a potential contributor to the metabolic benefits of bariatric surgery [57] , [58] , [59] . We investigated whether intestinal FGF15 modulates shifts in the microbial communities by VSG. To determine the effects of FGF15 on VSG-induced gut microbiota alteration, we performed 16S ribosomal RNA (rRNA) gene sequencing on cecal content samples collected 12 weeks after surgery (collected at the time of sacrifice). Chao1 and Shannon index were used to estimate with-in sample richness and diversity, respectively. The former represents the total number of microbes present in one single sample, while the latter accounts for both richness and evenness of the microbes. We did not see significant changes in richness (Chao1 index) and diversity (Shannon index) (Fig. 7a, b ). However, there was a trend toward increased richness in both VSG groups compared to their respective Sham controls. In addition, we observed a trend of decreased cecal diversity in FGF15 INT-KO Sham compared to Control Sham mice (Fig. 7b ). Fig. 7: Intestinal FGF15 modulates microbiota in cecal content. a Chao1 abundance and b Shannon index diversity of the gut microbiota in the cecal contents. LEfSex analysis depicting nodes within the bacterial taxonomic hierarchy that are enriched in cecal microbiota from c Control Sham versus FGF15 INT-KO Sham and d Control Sham versus VSG and e FGF15 INT-KO Sham versus VSG. Diagrams generated by LEfSe indicating differences at phylum , order , class , family , and genus levels between the two groups. f Top-ranked taxa at genus level identified by random forest analysis according to their ability to discriminate the microbiota of Sham and VSG mice per genotype in decreasing order of discriminatory importance. A comparison of the abundance of markers in VSG relative to Sham counterparts in each genotype. g . Differences in relative abundance of taxa at genus level. Animal number Control Sham ( n = 6), Control VSG ( n = 7), FGF15 INT-KO Sham ( n = 7), FGF15 INT-KO VSG ( n = 5). Data in ( a , b ) are shown as means ± SEM. * p < 0.05 (two-way ANOVA with Tukey’s post hoc test). Full size image Linear discriminant analysis (LDA) effect size (LEfSe) analysis showed taxonomic differences in the microbiota composition of the cecal content between Control Sham and FGF15 INT-KO Sham groups (Fig. 7c ). Firmicutes and Bacteroidetes are the most abundant phyla in fecal microbiota. The relative proportion of Firmicutes and Bacteroidetes has been reported to be affected differently by obesity and high-fat feeding Firmicutes at the phylum level, Erysipelotrichales at order level, and Allobaculum and Ruminococcus at the family level showed a trend of decreased abundance in FGF15 INT-KO Sham compared to Control Sham (Supplementary Fig. 8b, e, h, i ). However, Lachnospiraceae at the family level and Bacteroides at the genus level were increased in FGF15 INT-KO Sham compared to Control Sham (Supplementary Fig. 8f, g ). LDA effect size (LEfSe) analysis showed taxonomic differences in the microbiota composition of the cecal content between Sham and VSG in both genotype groups (Fig. 7d, e ). To further define bacteria characteristic of enrichment of Sham and VSG in each genotype, we also performed a random forest model. Lactobacillus species have been suggested to confer beneficial effects in a broad spectrum [60] , [61] . At the genus level, Lactobacillus , with an importance score of 0.301 determined by the decrease in the classification accuracy when it was ignored, was identified as the top-ranked discriminator for the Control VSG compared to Control Sham gut microbiota. On the other hand, Enterococcus genus was identified as the top discriminator for FGF15 INT-KO VSG vs. FGF15 INT-KO Sham gut microbiota, with Lactobacillus genus having an importance score of 0.088. (Fig. 7f, g ). Increased circulating bile acids are one of the hallmarks of bariatric surgery, and our group and others have identified bile acid signaling through FXR as a molecular link mediating the beneficial metabolic effects of elevated bile acids following VSG [12] , [13] . Secretion of FGF15/19 is a key response to FXR activation. Consistent with human data that show increased circulating levels of FGF19 after bariatric surgery [22] , [32] , [33] , [38] , [39] , [40] , VSG in mice upregulates FGF15 expression in the ileum (Fig. 1 ). Here we demonstrate that intestinal FGF15 is necessary for many of the metabolic, morphologic, and microbiome responses to VSG. To study the specific role of intestinal FGF15 in the response to VSG, we built a mouse model that allowed for specific deletion of FGF15 from the intestine in the adult animal (see Fig. 1 and “Methods”). Compared to control animals, these mice have similar body weight, body fat, food intake, and glucose regulation when challenged on a HFD. These data argue that intestinally derived FGF15 is not necessary for physiologic regulation of energy balance and glucose levels in diet-induced obese animals without bariatric surgery. It is important to note that these findings differ from gut-specific ablation of FXR, findings that were hypothesized to be dependent upon FXR’s downstream target FGF15 [62] , [63] . Gut-specific FXR knock out mice (VilCre; FXR flox/flox) are metabolically fit and resistant to HFD-induced metabolic disease [63] , [64] . However, ablation of FXR in adult mice (VilCreERT2; FXR flox/flox) does not lead to resistance to HFD-induced obesity, similar to our FGF15 INT-KO Sham mice [13] . It is also important to note that we previously found that unlike wild-type mice, FXR−/− mice did not maintain body weight loss and did not have improved glucose tolerance after VSG and while maintained on HFD [12] . A caveat of these studies is that FXR−/− mice are resistant to HFD-induced obesity and glucose intolerance, and therefore, the window for improvement in these parameters is smaller [65] . This is also the case for total body FGF15−/− mice, as we also recently reported [43] . The key point is that it is likely that FXR and FGF15’s role in metabolic regulation is different in various tissues and it is also sensitive to ablation during development versus in the adult mouse. These are critical components for interpreting the role bile acid metabolism plays following bariatric surgery and a major rationale for why we built a model that would allow for tissue-specific deletion of FGF15 in the adult mouse. Once released from the ileum, FGF15 enters the portal venous circulation and travels to the liver where FGF15 binds to its receptor FGFR4 and represses de novo bile acid synthesis through suppression of the rate-limiting enzyme cholesterol 7a-hydroxylase ( Cyp7a1 ) [14] . Therefore, bile acids and FGF15/19 inhibit further bile acid synthesis and facilitate communication between the small intestine and liver. As predicted, the lack of FGF15 resulted in increased plasma bile acids and cecal bile acid content in FGF15 INT-KO Sham mice (Fig. 6 ). After VSG, plasma bile acids were further increased in FGF15 INT-KO VSG mice, but cecal bile acids levels were suppressed (Fig. 6 ). This suggests that VSG directly alters the compartmental-specific bile acid pool independently of FGF15. Patients with NAFLD have increased hepatic Cyp7a1 levels [22] . Exogenous administration of FGF19 and its analog NGM282 did not correct hyperglycemia in diabetic patients, but caused a rapid and sustained reduction in hepatic Cyp7a1 levels and liver fat content in NAFLD patients [22] . Consistent with these observations, we saw increased hepatic expression of Cyp7a1 in FGF15 INT-KO Sham mice compared to Control Sham (Fig. 6 ). However, hepatic Cyp7a1 was significantly downregulated in FGF15 INT-KO VSG (Fig. 6 ). We speculate that the drastic increase in plasma bile acid levels in FGF15 INT-KO VSG mice downregulates hepatic Cyp7a1 expression as a negative feedback independent of circulating FGF15 [66] , [67] . The reduction of hepatic Cyp7a1 in FGF15 INT-KO VSG mice is VSG-dependent and FGF15-independent (unlike observed in FGF15 INT-KO Sham). As there are higher levels of cholesterol, bile acid synthesis is facilitated because there is more substrate. However, Cy7a1 is high in the FGF15 INT-KO Sham, because in the absence of FGF15 there is less to inhibit de novo synthesis. But, for FGF15 INT-KO VSG, the high amount of hepatic cholesterol and decreased hepatic bile acid uptake (decreased expression of Slc10a1 (coding for Ntcp and Oatp4 ), leads to high plasma bile acids, creating negative feedback, and as a result Cyp7a1 is downregulated in the FGF15 INT-KO VSG. Decreased hepatic Slc10a1 and Oatp4 and normal hepatic bile acid levels suggest that the liver is actively reducing bile acid uptake, leaving increased plasma bile acid pool. FGF15 INT-KO VSG mice have very high bile acids levels in plasma, but not in feces. This is consistent with FGF15 INT-KO VSG mice having increased recycling of bile acids compared to FGF15 INT-KO Sham. Ileal expression of Slc10a2 (coding for Asbt) trended higher in FGF15 INT-KO VSG compared to FGF15 INT-KO Sham, which would lead to better reabsorption in the ileum, and decreased fecal bile acids. We speculate that if the bile acid recycling is higher in FGF15 INT-KO VSG, then there is no need to produce more bile acids, and therefore hepatic Cyp7a1 expression decreases. Further understanding of the mechanisms that suppress Cyp7a1 would also be useful for cancer treatments that aim to block FGFR4 [68] . FGF15/19 signaling has been implicated in the development of hepatocellular carcinoma, making FGFR4 antagonists attractive candidates for treating this disease [68] . However, blockade of FGFR4 signaling inhibits the FGF15/19-induced bile acid brake. The resulting elevation in hydrophobic bile acids, as seen in FGF15 INT-KO VSG mice, act as detergents and disrupt cell membranes, and can lead to liver damage [69] . Although we see significantly elevated levels of plasma bile acids and very high levels of hydrophobic bile acids (Fig. 6 and Supplementary Fig. 6 ) in the FGF15 INT-KO VSG compared to Control VSG mice, we do not observe signs of liver damage as noted by normal circulating levels of ALT in FGF15 INT-KO VSG mice (Fig. 5 ). Our data also found that intestinal FGF15 is necessary for the reduction in hepatic cholesterol content after VSG. FGF15 INT-KO VSG mice had increased liver weight (normalized to body weight), despite decreased hepatic glycogen content (Fig. 5 and Supplementary Fig. 4 ). Although plasma cholesterol levels were decreased in both groups after VSG, FGF15 INT-KO VSG mice had increased hepatic total and esterified cholesterol levels (Fig. 5 ). The cholesterol synthesis rate-limiting gene, Hmg-CoA reductase ( Hmcgr ), was upregulated in FGF15 INT-KO Sham compared to Control Sham mice, but surprisingly reduced after VSG in FGF15 INT-KO VSG mice (Fig. 5 ). Hepatic cholesterol efflux pump-ATP-binding cassette, sub-family G, members 5 and 8 ( Abcg5 and Abcg8 ) expression was decreased in FGF15 INT-KO VSG mice (Fig. 5 ). These data suggest that despite decreased cholesterol synthesis there is attenuated cholesterol export leading to elevated liver cholesterol content in FGF15 INT-KO VSG mice. FGF21 levels were increased in FGF15 INT-KO mice (especially after VSG; Supplementary Fig. 2 ). FGF21 levels are tighly linked to nutrional status, and it has been well established that FGF21 levels increase in fasting and after ketogenic and low-protein diets [70] , [71] , [72] . The lack of FGF15, which is a postprandial hormone, could be altering the gut-liver communication and leading to the liver sensing a “fasting state” and increasing FGF21 levels [73] . Clinical and mouse studies have reported increased plasma FGF21 levels in patients and animal models of NAFLD [74] , [75] , [76] . Consistent with these data, we hypothesize that plasma FGF21 is increased in FGF15 INT-KO mice as compensatory mechanism to attenuate liver injury and hepatic lipid accumulation [77] . Importantly, we did not observe increased hepatic cholesterol levels in FGF15 INT-KO Sham mice compared to Control Sham (despite increased hepatic expression of Hmcgr ). It is possible that the hepatic cholesterol in these mice is directed towards their increased plasma bile acid levels. It is also possible that increased FGF21 levels in FGF15 INT-KO Sham were sufficient to counteract the hepatic lipid accumulation and liver damage. Alternatively, other tissues, including muscle and adipose tissue, could be responsible for the increased FGF21 levels in FGF15 INT-KO VSG mice [78] . This is consistent with the observation that elevated plasma FGF21 levels have been linked to decreased muscle mass [50] and reduced bone mineral density and BMAT [79] , [80] , [81] . Taken together these observations point to the possibility that plasma FGF21 levels are not a mediator of the profound cachexia observed in FGF15 INT-KO VSG mice and are increased in response to the muscle mass loss and/or hepatic lipid accumulation in these mice. We did not find a difference in glucose excursion between Control Sham and FGF15 INT-KO Sham mice, suggesting that intestinal-derived FGF15 does not play an essential role in peripheral glucose tolerance, at least under HFD conditions (Fig. 4 ). As expected, we saw an improvement in glucose tolerance in Control VSG compared to Control Sham mice after intraperitoneal glucose challenge (ipGTT; Fig. 4 ). To our surprise, there was no difference in glucose tolerance between FGF15 INT-KO VSG and FGF15 INT-KO Sham mice, despite the large body weight loss in FGF15 INT-KO after VSG (Fig. 4 ). Loss in muscle mass as seen in FGF15 INT-KO VSG can greatly inhibit the proper disposal of glucose, leading to glucose intolerance. However, VSG in total body FGF15−/− mice also did not improve glucose tolerance despite lack of change in lean tissue mass, suggesting that these effects are FGF15-dependent and body weight-independent [43] . In addition, gallbladder bile diversion to the ileum, a surgical procedure that also results in sustained weight loss and improved glucose tolerance, is ineffective in restoring glucose tolerance in gut-specific ablation of FXR in adult mice [13] . Taken together, these data support the conclusion that the lack of improvement in glucose tolerance in our FGF15 INT-KO mice is dependent upon the enterohepatic system. Recent studies reported that patients who experience post-bariatric postprandial hypoglycemia have increased postprandial levels of FGF19, linking the levels of FGF15/19 to glucose regulation after weight-loss surgery [38] . It has been reported that reduced expression of FGF15 in mice is associated with increased gastrointestinal motility and increased luminal water content, similar to human bile acid diarrhea [82] . However, gastric emptying was lower in FGF15 INT-KO Sham compared to Control Sham mice (Fig. 4 ). We speculate that the decrease in gastric emptying is a result of increased circulating bile acids in FGF15 INT-KO Sham mice, especially increased TDCA or DCA levels [83] . These differences in gastric emptying rates change after VSG. FGF15 INT-KO VSG had increased gastric emptying compared to Control VSG mice (Fig. 4 ). Consistent with previous reports, we also saw an increased total GLP-1 postprandial response in Control VSG mice after a mixed meal. The increase in total GLP-1 after VSG has been attributed to the rapid entry of ingested glucose and nutrients into the small intestine [84] . However, the GLP-1 (basal and postprandial) in FGF15 INT-KO VSG mice were much higher than Control VSG (Fig. 4 ). This points to a more complicated regulation of GLP-1 secretion beyond simply nutrient presentation. Strong evidence links bile acid activation of TGR5 to increased GLP-1 secretion [85] , [86] , [87] . Consequently, elevated levels of plasma bile acids, such as TLCA (TGR5 agonist), in FGF15 INT-KO mice given VSG may act to increase TGR5 signaling and drive increased GLP-1 secretion [88] . Interestingly, despite the elevated GLP-1 levels, FGF15 INT-KO mice given VSG do not have improved glucose tolerance pointing to a potentially more critical role of FGF15 as compared to GLP-1. One of the most profound and surprising findings was that FGF15 INT-KO mice lose considerably more weight than the control mice after VSG (Fig. 1 ). While we have consistently observed that mice given a VSG lose little or no lean mass [48] , [89] , FGF15 INT-KO lose 25% of their lean tissue, much more than the control VSG mice (Fig. 1 ). Thus, while FGF15 does not mediate reductions in body fat after VSG, it is essential to protect from deleterious loss of lean mass after VSG. Loss of muscle mass is a major concern in the setting of rapid weight loss interventions such as very-low-calorie diets and bariatric surgery [90] , [91] , [92] , [93] . A second component of cachexia in the FGF15 INT-KO VSG mice was due to reduced bone mass and BMAT (Fig. 2 ). Bariatric procedures including VSG can result in bone loss beyond the normal response to reduced loading from weight loss, or calcium deficiency from diminished absorption [52] , [90] , [94] . In FGF15 INT-KO mice this effect of surgery is amplified and results in a diffuse pattern of osseous abnormality including both trabecular and cortical bone mass and BMAT (Fig. 2 ). In humans, reduction in bone density after bariatric surgery can predispose to fractures and is an important downside to the use of these procedures [90] . It remains to be seen whether this post-surgical metabolic bone disease can be accounted for by FGF15/19 signaling as suggested by our findings. The cachexia observed in FGF15 INT-KO mice after VSG was surprising and we sought to identify potential mechanisms for the dramatic loss in muscle and bone mass in these mice. Fibroblast growth factor 23 (FGF23), the third member of the endocrine FGFs (in addition to FGF15/19 and FGF21), is a bone-derived hormone that regulates mineral homeostasis and consequently bone mineral density [54] , [56] . Plasma FGF23 levels were dramatically elevated in FGF15 INT-KO VSG mice (Fig. 3 ). Next, to investigate the source of increased plasma FGF23 levels, we measured circulating erythropoietin (EPO), a known driver for increased FGF23 and bone loss [55] , [56] . Further, elevated EPO is also sufficient to stimulate loss of bone and BMAT [95] . EPO was also highly increased in FGF15 INT-KO VSG mice (Fig. 3 ). Plasma phosphate and 25 (OH) vitamin D levels were unaffected, as has been reported in mice overexpressing EPO and high plasma FGF23 levels despite bone loss [54] . We were intrigued by these findings as increased plasma FGF23 and EPO levels are often observed in anemia. We have previously reported lower iron levels are observed in bariatric surgeries with widely varying impacts on duodenal exposure to chime, including VSG [96] . Hemoglobin levels were decreased in FGF15 INT-KO VSG compared to FGF15 INT-KO Sham mice, but ferritin levels were unaffected (Fig. 3 ). Both VSG mice trended toward increased iron levels in cecal contents but these were not FGF15-dependent. An increase in circulating EPO but normal ferritin levels and near compete depletion of BMAT, suggest that FGF15 INT-KO VSG mice have bone marrow dysfunction leading to anemia of chronic disease. Our previous studies have shown that loss of bone mass and BMAT after VSG is inversely correlated with myeloid cell expansion in marrow [52] . Therefore, the mechanism for these unexpected findings has to be a factor dependent on both FGF15 and VSG. FGF15 INT-KO VSG mice had high levels of circulating hydrophobic bile acid levels (Fig. 6E , Supplementary Fig. 6 ). Hydrophobicity is an important factor for bile acid toxicity and cholestatic injury [97] , [98] . Therefore, we hypothesize that increased hydrophobic bile acids are an important contributor to the cachexia seen after VSG in FGF15 INT-KO mice (Fig. 8 ). The lack of gut-derived FGF15 is sufficient to increase circulating total bile acids (as can VSG), however, the combination of lack in gut FGF15 along with VSG results in very high levels of circulating total and most importantly, hydrophobic levels of bile acids (Fig. 6 ). Increase in circulating hydrophobic bile acids can lead to bile acid toxicity that may contribute to the cachexia observed in FGF15 INT-KO VSG mice. Further, VSG in total body FGF15−/− mice did not lead to cachexia consistent with relatively normal plasma levels of bile acids (compared to WT VSG) [43] . Fig. 8: Intestinal-derived FGF15 protects against deleterious effects following sleeve gastrectomy in mice. VSG leads to an increase in ileal expression of FGF15 and total plasma bile acids. In the absence of intestinally derived FGF15 (FGF15 INT-KO ), VSG leads to an even greater increase in circulating total and specifically, hydrophobic bile acids. We speculate that the increase in hydrophobic bile acids leads to bone marrow dysfunction, which increases EPO and FGF23 levels that likely contribute to potentially serious loss of bone mass, bone marrow adipose tissue (BMAT), inducing anemia of chronic disease. FGF15 INT-KO VSG mice have a loss of muscle mass and cardiac hypertrophy, as a result of bile acid toxicity or secondary to anemia of chronic disease. FGF15 INT-KO VSG mice also have increased hepatic cholesterol and they do not show improved glucose tolerance following VSG. Full size image Together, these data lead us to speculate that bile acids and bile acid toxicity is a critical contributor to the muscle and bone loss in FGF15 INT-KO VSG mice (Fig. 8 ). Recent study showed that antibiotic treatment and the resultant change in microbiota and intestinal bile acids results in skeletal muscle atrophy by decreasing bile acid-FXR-FGF15 signaling [99] . It has also been reported that exogenous FGF19 induces skeletal muscle hypertrophy and blocks muscle atrophy induced by glucocorticoid treatment, sarcopenia and obesity [49] . The mechanism behind these findings is not well understood, but bile acids may play a role. We also hypothesize that dramatic increases in EPO and FGF23 play a major role in bone density and BMAT loss in FGF15 INT-KO VSG mice. It remains unclear if and how bile acid toxicity induces anemia of chronic disease leading to the increase in EPO and FGF23. Further supporting the bile acid toxicity hypothesis, FGF15 INT-KO VSG mice have cardiac hypertrophy (Fig. 3 ). Elevated plasma bile acids that occur in mice with knock outs of both FXR and Shp or by pharmacological administration of the bile acids TCA and LCA also result in cardiac hypertrophy and reduced cardiac output [100] , [101] . In addition, anemia and increased FGF23 and EPO can also induce cardiac hypertrophy [102] , [103] . Future studies will dissect the effect of bile acid toxicity on the cardiovascular function of FGF15 INT-KO VSG mice, as these are important parameters for patients undergoing bariatric surgery procedures. The critical point from these studies is that VSG increases circulating levels of bile acids by a mechanism that remains unclear. Our data lead us to hypothesize that the increase in FGF15 after VSG serves as an important break to limit this increase so as not to become deleterious and lead to potentially toxic levels of bile acids. In the absence of intestinally derived FGF15, VSG leads to an even greater increase in hydrophobic bile acids which we speculate leads to anemia of chronic disease and increased EPO and FGF23 levels that likely contribute to great loss of bone mass, BMAT, muscle mass, and cardiac hypertrophy. Circulating levels of FGF19 increase in humans after VSG, but this increase is variable between patients [22] , [32] , [33] , [38] , [39] , [40] . Our data suggest that bariatric surgery patients with low FGF19 levels may be at a higher risk for bone and skeletal muscle loss as well as increased hepatic cholesterol accumulation. As with many studies using the mouse to model human effects, there are important caveats to the extrapolation to humans. Not all aspects of the regulation of enterohepatic circulation are identical in mouse and human and thus further work will be needed. These experiments are time and labor intensive so we have not directly tested whether lowering of plasma bile acids would prevent some deleterious effects of VSG in FGF15 INT-KO mice. Future work will directly address potential therapeutic strategies that could limit these deleterious effects of VSG. More research is warranted to determine if circulating FGF19 can act as a biomarker to identify patients that are at high risk for excessive bile acid levels and these negative outcomes following bariatric surgery. Understanding this relationship would allow physicians to optimize treatment strategies for at risk patients. Study approval All protocols complied with all relevant ethical regulations for animal testing and research. All protocols were approved by the University of Michigan (Ann Arbor, MI) Animal Care and Use Committees and were in accordance to NIH guidelines. Generation of FGF15 flox mouse Gene sequence for the mouse FGF15 gene (4.4k base pair double strands DNA containing fgf15 exon) was downloaded from genebank. Guide RNAs were designed against the mouse sequence containing the region of interest for targeting (introns flanking FGF15 exon 2) using prediction algorithms available through http://crispor.tefor.net/ . Guides were selected based on the specificity score and predicted efficiency (Mor.Mateos). Selected single guide RNA (sgRNA) sequences were subcloned into plasmid pX330 and subsequently confirmed by sequencing. Targeting DNA oligonucleotides including the 34 base pairs loxP site and 81-82 nucleotides of flanking sequence on either side were generated (IDT Technologies). DNA oligonucleotides were designed to disrupt the sgRNA and PAM sequences so that Cas9 would not be able to cleave the inserted sequence after incorporation into the genome. To test the ability of the sgRNAs to cut chromosomal DNA appropriately, each sgRNA was injected into fertilized eggs by the University of Michigan Transgenic Animal Core; zygotes were then allowed to develop into blastocysts in culture. PCR amplification of the target region followed by sequencing was used to confirm Cas9 dependent DNA cutting in vivo. Cas9/sgRNA/oligo donor were then injected into 300 fertilized mouse eggs (C57BL/6x SJL) and transferred to pseudo-pregnant recipients for gestation. After delivery of potential founders, tail DNA was isolated and screened by PCR across the region of interest to identify genomic manipulations. As founders are often mosaic for allelic changes, PCR products of genomic DNA were subcloned into topo vector and sequenced to characterize the genetic modification in the mice. Animals and diet The FGF15 flox/flox mice, were built using CRISPR-Cas9 technology with LoxP sites flanking exon 2 of the FGF15 gene (described above). We bred these mice to VilCreERT2 mice (C57BL background) and administered tamoxifen (intraperitoneal, 3 doses/150 mg/kg) to VilCreERT2; Fgf15 flox/flox and controls (VilCreERT2 and Fgf15 flox/flox). We validated exon 2 excision within the latter jejunal and ileal mucosa, where FGF15 is most highly expressed (Supplementary Fig. 1 ). Male mice (6–8 weeks of age) were single-housed under a 12-h light/dark cycle with ad libitum access to water and food. A week after tamoxifen administration, FGF15 INT-KO and Control male mice (all littermates) were placed on 60% HFD from Research Diets, Inc. (New Jersey, US; Catalog D12492) for 8 weeks. Mice were singly-housed under a 12-h light/dark cycle in a facility maintained at 25 °C with 50–60% humidity for the duration of the studies. Mice underwent VSG or Sham surgery (described below) and returned to 60% HFD four days after surgery until the end of the study. Animals were euthanized 12 weeks post-surgery (26-28 weeks of age). One Control Sham mouse died accidentally during NMR measurements on the day before necropsy. The post-necropsy data on metabolites and tissue gene expression for this Control Sham mouse was excluded, but the data not sensitive to nutritional state was included. The rest of the mice were fasted overnight, administered oral mixed meal (volume 200 µl Ensure Plus spiked with a 40-mg dextrose), and sacrificed 90 min later. Plasma and tissues were collected and frozen immediately. All animals were euthanized using CO 2. VSG in mice Mice were maintained on a 60% HFD for 8 weeks prior to undergoing Sham or VSG surgery [48] , [104] , [105] . Mice were fasted overnight prior to day of surgery. Animals were anesthetized using isoflurane, and a small laparotomy incision was made in the abdominal wall. The lateral 80% of the stomach along the greater curvature and fundus was excised in VSG animals by using an Echelon Flex TM powered vascular stapler (Ethicon Endo-Surgery, USA). The Sham surgery was performed by the application of gentle pressure on the stomach with blunt forceps for 15 seconds. All mice received one dose of Buprinex (0.1 mg/kg) and Meloxicam (0.5 mg/kg) immediately after surgery. All mice received Meloxicam (0.5 mg/kg) for 3 days after surgery and Enrofloxacin (40 mg/kg) for 5 days after surgery. Animals were placed on DietGel Boost (ClearH 2 O; Postland ME) for 3 days after surgery. They were placed back on pre-operative solid diet (60% HFD) on day 4 post-surgery. Body weight and food intake as well as overall health were monitored daily for the first 7 days after surgery and once weekly until end of the studies. Metabolic studies Body weight was monitored monthly for 9 weeks prior and 12 weeks after Sham/VSG surgery. Intraperitoneal glucose tolerance test (IPGTT) was performed by intraperitoneal (IP) injection of 50% dextrose (2 g/kg) in 4-h fasted mice. Mixed-meal tolerance test (MMTT) was performed via an oral gavage of liquid meal (volume 200 µl Ensure Plus spiked with a 40-mg dextrose and 4-mg acetaminophen, Sigma-Aldrich) in 4-hour fasted mice. Blood was obtained from the tail vein and blood glucose was measured with Accu-Chek blood glucose meter (Accu-Chek Aviva Plus, Roche Diagnostics). Blood was collected from the tail vein at baseline and 15 min after gavage in EDTA-coated microtubes. Plasma acetaminophen levels were used to assess the rate of gastric emptying and were measured using spectrophotometry assay (Sekisui Diagnostics). ELISA and metabolite assays Insulin (Crystal Chem), total GLP-1 (MesoScale Discovery), and acetaminophen (Sekisui Diagnostics) were measured during experiments shown in Fig. 3 . Insufficient amount of blood was obtained from one Control VSG for insulin, total GLP-1 and acetaminophen levels at 15 min. Postprandial plasma obtained at termination of studies (see above for details) was used to measure IGF-1 (R&D Systems), Activin-A (R&D Systems), Myostatin (GDF8) (R&D Systems), FGF21 (R&D Systems), L-amino acids (Abcam), Erythropoietin (Abcam), FGF23 (Abcam), Ferritin (Abcam), Hemoglobin (Abcam), Phosphate (Abcam), 25(OH) Vitamin D (Abcam). Iron levels in cecal contents were measured with Iron Assay Kit (Abcam). Glycogen content was measured in liver and muscle (tibialis anterior) samples with Glycogen Assay kit (Sigma-Aldrich). All sampled blood was collected via tail vein in EDTA-coated tubes. All assays were performed according to the manufacturer’s instructions. Plasma bile acid composition Plasma bile acid composition was measured by the University of Michigan Metabolomics Core using two-step solvent extraction. Supernatants are combined, dried, and re-suspended for LCMS separation by RPLC and measurements by ESI - QQQ MRM methods [106] . Sample preparation : 20 µL plasma was transferred to a microtube. Eighty microliters of chilled acetonitrile with 5% NH 4 OH, containing isotope-labeled internal standards was added to the tube, and the mixture vortexed until completely homogenized. The mixture was incubated on ice for 10 min and vortexed to remix. This homogenized mixture was centrifuged and 3 µL of the supernatant from each sample was removed to create a pooled sample for QC purposes. Next, 90 µL of the supernatant transferred to an LC-MS autosampler insert and brought to dryness in a speedvac set to 45 °C for ~45 min. Each sample was reconstituted in 100 µL of 50/50 Methanol/Water. A series of calibration standards ranging from 0 to 1000 nM were prepared along with samples to quantify metabolites. LC-MS analysis : LC-MS analysis was performed on an Agilent system consisting of a 1290 UPLC module coupled with a 6490 Triple Quad (QqQ) mass spectrometer (Agilent Technologies, Santa Clara, CA) operated in MRM mode. MRM transitions are included in the table below. Metabolites were separated on a 100 mm × 2.1 mm Acquity BEH UPLC (1.7 µm) column (Waters Corp, Milford, MA) using H 2 O, 0.1% Formic acid, as mobile phase A, and Acetonitrile, 0.1% Formic acid, as mobile phase B. The flow rate was 0.25 mL/min with the following gradient: linear from 5 to 25% B over 2 min, linear from 25 to 40% B over 14 min, linear from 40 to 95% B over 2 min, followed by isocratic elution at 95% B for 5 min. The system was returned to starting conditions (5% B) in 0.1 min and held there for 3 min to allow for column re-equilibration before injecting another sample. The mass spectrometer was operated in ESI- mode according to previously published conditions. Data were processed using MassHunter Quantitative analysis version B.07.00. Metabolites were normalized to the nearest isotope-labeled internal standard and quantitated using two replicated injections of five standards to create a linear calibration curve with accuracy better than 80% for each standard. Using ROUT method and treating all the values in all subgroups as one set of data ( Q = 1), we identified three samples (one Control VSG and two FGF15 INT-KO Sham) as significant outliers. QQ plot and Homoscedasticity plot showed that these samples were out of the normal distribution. In addition, analysis of total bile acids in the same samples using Total Bile Assay (NBT Method) (GenWay Biotech Inc; San Diego, CA) also revealed that these samples are abnormally elevated. Therefore, these samples were excluded from all plasma bile acid data analysis. Plasma bile acid composition data are available at the NIH Common Fund’s National Metabolomics Data Repository (NMDR) website, the Metabolomics Workbench, https://www.metabolomicsworkbench.org where it has been assigned Project ID (PR001116). The data can be accessed directly via it’s Project DOI: (10.21228/M8FM51). Lipid and bile acid measurements in tissues Liver and cecal content lipids were extracted using Lipid Extraction Kit Chloroform Free (Abcam). Total and cholesterol ester (Millipore/Sigma-Aldrich), triglycerides (Abcam), free fatty acids (Abcam), and total bile acids (Total Bile Assay (NBT Method), GenWay Biotech Inc; San Diego, CA) were measured using the extracted liver lipids. Cecal content total bile acids were measured using the extracted cecal content lipids (Total Bile Assay (NBT Method) assay, GenWay Biotech Inc; San Diego, CA). Postprandial plasma obtained at termination of studies (see above for details) was used to measure total cholesterol (Pointe Scientific), triglycerides (Pointe Scientific), free fatty acids (Abcam), ALT (Pointe Scientific). All assays were performed according to the manufacturer’s instructions. Bone parameters Tissues were fixed in 10% neutral-buffered formalin for 24 h and kept in Sorenson’s buffer (pH7.4) thereafter. Tibiae were placed in a 19-mm diameter specimen holder and scanned over the entire length of the tibiae using a microcomputed tomography (μCT) system (μCT100 Scanco Medical). Scan settings were as follows: voxel size 12 μm, 70 kVp, 114 μA, 0.5 mm AL filter, and integration time 500 ms. Density measurements were calibrated to the manufacturer’s hydroxyapatite phantom. Analysis was performed using the manufacturer’s evaluation software and a threshold of 180 for trabecular bone and 280 for cortical bone. Tibiae used for μCT scanning were decalcified in 14% EDTA for 3 weeks. Paraffin-embedded tissue sections were processed and stained with H&E. Bone Marrow Adipose Tissue Quantification by Osmium Tetroxide Staining and μCT: Mouse tibiae were decalcified in 14% EDTA for 2-3 weeks, and then put into 1% osmium tetroxide solution (diluted by Sorenson’s buffer pH7.4) for 48 h. Osmium tetroxide-stained bones were scanned by the same program as described above. A threshold of 400 Gy was used for BMAT quantification. The volume of BMAT was normalized by the total volume (TV) of bone and shown as percentage (%). Muscle fiber area and ileal crypt depth/villi height analysis Soleus muscle and ileal section were dissected and fixed in 10% neutral-buffered formalin overnight. Tissue was embedded in paraffin and sectioned onto slides and stained for H&E following standard protocol. Photos, and analysis of muscle fiber area (in 100–250 muscle fibers), and ileal crypt depth, and ileal villi height (in 25 villi and crypts) were acquired using Olympus IX73 fluorescence microscopy system (Olympus). Villus height was measured from the crypt-villus junction to the tip of the villus and crypt depth was measured from the base of the crypt to the crypt-villus junction. Images were analyzed using Olympus cellSens Standard imaging software (Olympus). Grip strength Grip strength was measured with Columbus Instruments Grip Strength Meter (Colombus Instruments), which assesses neuromuscular function by sensing the peak amount of force an animal applies in grasping specially designed pull bar assemblies. Metering was performed with precision force gauges in such a manner as to retain the peak force applied on a digital display. The dual sensor model was employed by first allowing the animal to grasp the forelimb pull bar assembly. The animal was then drawn along a straight line leading away from the sensor. The animal released at some point and the maximum force attained is stored on the display. Each animal was tested five times and the average force reported in the data. Grip strength test was performed by the University of Michigan Physiology Phenotyping Core. Absorbed energy content Fecal energy was assessed by the University of Michigan Animal Phenotyping core using Bomb Calorimeter, Parr 6200, and 1108P oxygen bomb [107] . Mice were single-housed in clean housing cages for one week. Food weight was determined for the same time period. All fecal samples are collected using forceps and weighed to determine “wet weight”. Prior to processing, fecal samples are dried overnight at 50 °C. Samples are then removed from the oven one at a time and weighed. Sample weights are recorded and fecal samples are then ground-up individually. Samples are ground with mortar and pestle and carefully scooped into a dry tube. All instruments were washed with sparkleen and 10% bleach and completely dried between samples. New weigh boats are used for each sample and weighed on the same scale as the pre-dried weights. Quantitative real-time PCR RNA was extracted from tissue samples using RNeasy isolation kit (Qiagen). cDNA was synthesized by reverse transcription from mRNA using the iScript cDNA Synthesis Kit (Bio-Rad). 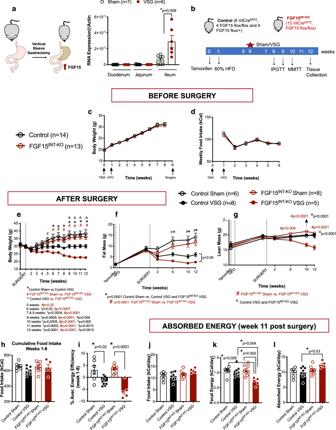Fig. 1: Intestinal FGF15 expression increases and prevents muscle mass loss after VSG in mice. aFGF15RNA expression in duodenum, jejunum and ileum in control Sham and VSG mice fed 60% HFD. Intestinal mucosa was collected 15 min post mixed meal gavage (n= 6 Sham and 7 VSG).bExperimental timeline.cBody weight anddfood intake before surgery.eBody weight after surgery.fFat body mass andglean body mass before and after surgery.hCumulative food intake andienergy efficiency for weeks 1–8 after surgery.jFood intake,kfecal energy andlabsorbed energy during week 11 after surgery. Animal number: Control Sham (n= 6), Control VSG (n= 8), FGF15INT-KOSham (n= 8), FGF15INT-KOVSG (n= 5). Data are shown as means ± SEM. Panelsa,c, anddwere analyzed with Student’s two-tailedttest. Panelse–lwere analyzed with two-way ANOVA with Tukey’s post hoc test. *p< 0.05. Gene expression was performed by quantitative real-time RT-PCR using Taqman gene expression assay (Supplementary Table 1 ) and was performed using StepOnePlus detection system (Applied Biosystems) with a standard protocol. Relative abundance for each transcript was calculated by a standard curve of cycle thresholds and normalized to RL32 . One Control VSG ileum sample was excluded due to the high cycle threshold of RL32 (Ct over 30 after two independent measurements). Intestinal biometry Following euthanasia, the entire gastrointestinal tract from the stomach to the rectum was removed, cleaned of mesenteric fat and gut weight and length determined. Small and large intestine/colon length was measured on a horizontal ruler after flushing with PBS. The entire small and large intestine/colon were then blotted to remove PBS before being weighed. Analysis of 16S rRNA Gene Sequences 16S rRNA Sequencing: Cecal contents were added to individual Bead plate provided by the Microbiome Core at the University of Michigan. DNA was isolated using Qiagen MagAttract PowerMicrobiome kit DNA/RNA kit (Qiagen, catalog no. 27500-4-EP) on the EpMotion 5075 (Eppendorf) liquid handler. Extracted DNA was then used to generate 16S rRNA libraries for community analysis. The DNA libraries were prepared by the Microbiome Core as described previously [108] . Briefly, DNA was PCR amplified using a set of barcoded dual-index primers specific to the V4 region of the 16S rRNA gene [109] . PCR reactions are composed of 5 µL of 4 µM equimolar primer set, 0.15 µL of AccuPrime Taq DNA High Fidelity Polymerase, 2 µL of 10x AccuPrime PCR Buffer II (Thermo Fisher Scientific, catalog no.12346094), 11.85 µL of PCR-grade water, and 1 µL of DNA template. The PCR conditions used consisted of 2 min at 95 °C, followed by 30 cycles of 95 °C for 20 s, 55 °C for 15 s, and 72 °C for 5 min, followed by 72 °C for 10 min. Each PCR reaction is normalized using the SequalPrep Normalization Plate Kit (Thermo Fisher Scientific, catalog no. A1051001). The normalized reactions are pooled and quantified using the Kapa Biosystems Library qPCR MasterMix (ROX Low) Quantification kit for Illumina platforms (catalog no. KK4873). The Agilent Bioanalyzer is used to confirm the size of the amplicon library (~399 bp) using a high-sensitive DNA analysis kit (catalog no. 5067-4626). Pooled amplicon library is then sequenced on the Illumina MiSeq platform using the 500 cycle MiSeq V2 Reagent kit (catalog no. MS-102-2003) according to the manufacturer’s instructions with modifications of the primer set with custom read 1/read 2 and index primers added to the reagent cartridge. The “Preparing Libraries for Sequencing on the MiSeq” (part 15039740, Rev. D) protocol was used to prepare libraries with a final load concentration of 5.5 pM, spiked with 15% PhiX to create diversity within the run. FASTQ files are generated when the 2 × 250 bp sequencing completes. Analysis: Following sequencing, microbiome bioinformatics were run using QIIME 2 2020.2 [110] . Briefly, non-singleton amplicon sequence variants (ASVs, 100% operational taxonomic units (OTUs)) were generated from raw sequences after trimming with the cutadapt plugin denoising with the dada2 plugin. One Control VSG and one FGF15 INT-KO Sham samples were excluded because of low OTUs. Taxonomy was then assigned to ASVs using the classify-sklearn alignment algorithm (Bokulich et al. [111] ) against the Greengenes database (Release 13.8) of 99% OTUs reference sequences (McDonald et al. [112] ). 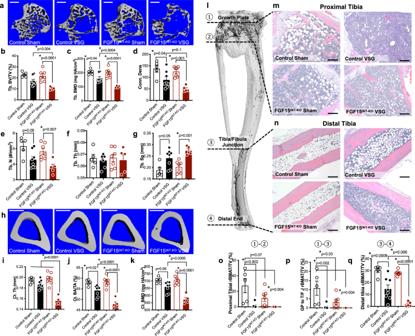Fig. 2: Intestinal-derived FGF15 partially preserves bone and bone marrow adipose tissue (BMAT) loss following VSG. a3D images of trabecular bone, scale bars 500 μm.bTrabecular bone volume fraction (Tb. BV/TV),ctrabecular bone mineral density (Tb. BMD),dtrabecular bone connective density (Conn. Des) andetrabecular number (Tb. N),fthickness of the trabecular bone (Tb. Th),gspacing between trabeculae (Tb. Sp).h3D images of mid-cortical bone, scale bars 500 μm.iThickness of the cortical bone (Ct. Th).jCortical bone area (Ct. BA/TA) andkcortical bone mineral density (Ct. BMD).lTibial BMAT was visualized by osmium staining.m,nRepresentative sections from proximal and distal tibiae were stained with H&E and are shown at ×100 magnification, scale bars 200 μm.lTibial BMAT was quantified relative to total bone volume after osmium staining within the indicated regions as shown in (o) proximal Tibia (①-②),pgrowth plate (G/P) to tibia/fibula junction (T/F J) (①-③),qdistal tibia is T/F J to distal end (③-④). Animal number: Control Sham (n= 5), Control VSG (n= 8), FGF15INT-KOSham (n= 7), FGF15INT-KOVSG (n= 5). Data are shown as means ± SEM. *p< 0.05 (two-way ANOVA with Tukey’s post hoc test). Alpha diversity metrics including Chao1 and Shannon, which estimate with-in sample richness and diversity respectively, were calculated using the diversity plugin. Chao1 index represents the number of ASVs present in one single sample, while Shannon index accounts for both abundance and evenness of ASVs present. Beta diversity metrics including weighted and unweighted UniFrac distance matrix [113] , which estimate between-sample dissimilarity, were scaled and visualized through principal coordinates analysis (PCoA), and further used to determine the significance of the clustering between groups via permutational multivariate analysis of variance (PERMANOVA). Linear discriminant analysis (LDA) effect size (LEfSe) with default parameters [114] and Random Forest Classifier (QIIME 2 2020.2) with 10-fold cross-validations [115] were computed to identify significantly different microbes in abundance between groups at different taxonomic levels. The 16S rRNA Sequencing composition data generated in this study have been deposited in the Sequence Read Archive (SRA) where it has been assigned BioProject ID PRJNA734599. The data can be accessed directly via it’s Project URL: http://www.ncbi.nlm.nih.gov/bioproject/734599 . Statistics and reproducibility The researchers were blinded during studies and mouse order (per genotype and surgery) were randomized. Microcomputed tomography (μCT) analysis for bone parameters and bone marrow adiposity were completed by two independent experienced lab researchers in a blinded manner. Bone histology images were taken from each individual mouse and all images were quantified. 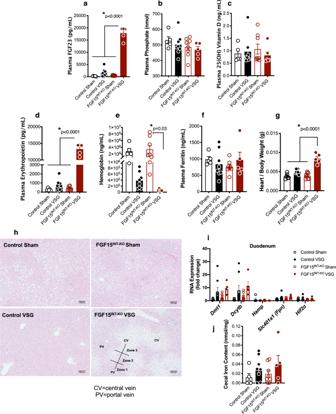Fig. 3: Loss of intestinal FGF15 increases circulating fibroblast growth factor 23 (FGF23) and erythropoietin (EPO) levels after VSG. Plasma levels ofaFGF23,bphosphate,c25(OH) vitamin D,derythropoietin,ehemoglobin andfferritin.gHeart to body weight ratio.hH&E stain of liver sections, CV = central vein, PV = portal vein, Zones 1–3, scale bars 100 μm.iRNA expression ofDmt1, Dcytb,Hamp,Slc401a1(Fpn) andHif2αin duodenum.jIron levels in cecal contents. Animal number for (a–f) and (i,j): Control Sham (n= 5), Control VSG (n = 8), FGF15INT-KOSham (n= 8), FGF15INT-KOVSG (n= 5). Animal number for g: Control Sham (n= 6), Control VSG (n= 8), FGF15INT-KOSham (n = 8), FGF15INT-KOVSG (n= 5). Data are shown as means ± SEM. *p< 0.05 (two-way ANOVA with Tukey’s post hoc test). Representative images of the mean number based on the quantification were shown in Fig. 2 . Liver histology images were taken from each individual mouse and representative images were shown in Fig. 3 . All metabolic studies were performed at least twice with the same results and data were shown over multiple time points (body weight, body composition, food intake, glucose tolerance). All studies were performed in a sufficient number of biological replicates per genotype and surgery. Statistical analysis The statistical analysis for comparisons between two groups was performed by unpaired (two-tailed) Student’s t test. Two-way ANOVA with post hoc Tukey’s multiple comparisons post hoc test was used for comparisons among four groups. P values <0.05 were considered significant. Statistical analysis was performed using GraphPad Prism 8.2.0. Microbiome analysis is described above. 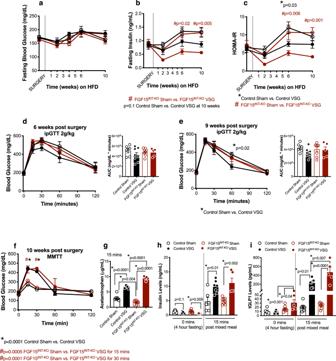Fig. 4: FGF15INT-KOmice remain glucose intolerant despite significant body weight loss after VSG. aFasting (4 h) blood glucose,bfasting (4 h) insulin levels andcHOMA-IR after surgery.dIntraperitoneal glucose tolerance test (ipGTT; 2 g/kg) performed 6-weeks post-surgery and Area Under the Curve (AUC).eIntraperitoneal glucose tolerance test (ipGTT; 2 g/kg) performed 9 weeks post-surgery and Area Under the Curve (AUC).fMixed meal tolerance test (MMTT) performed 10 weeks post-surgery.gGastric emptying rate measured by acetaminophen levels at 15 min post mixed meal.hInsulin levels at baseline (4 h fast) and 15 min post mixed meal.iTotal GLP-1 levels at baseline (4 h fast) and 15 min post mixed meal. Animal number (a–f) and (h,i): Control Sham (n= 6), Control VSG (n= 8), FGF15INT-KOSham (n= 8), FGF15INT-KOVSG (n= 5). Animal number g: Control Sham (n= 6), Control VSG (n= 7), FGF15INT-KOSham (n= 8), FGF15INT-KOVSG (n= 5). Data are shown as means ± SEM. *p< 0.05 (two-way ANOVA with Tukey’s post hoc test). 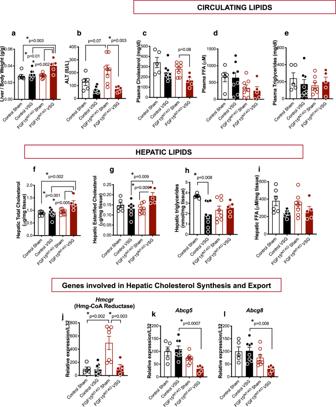Fig. 5: Loss of intestinal FGF15 results in aberrant hepatic lipid metabolism following VSG. aLiver weight normalized to body weight.bAlanine aminotransferase (ALT) plasma levels.cPlasma cholesterol.dPlasma-free fatty acids (FFA) andePlasma triglycerides (postprandial, 12 weeks post-surgery).fTotal hepatic cholesterol.gHepatic esterified cholesterol.hHepatic triglycerides.iHepatic free fatty acids. Hepatic RNA expression of cholesterol synthesis genej.Hmcgrand cholesterol export genesk.Abcg5andl.Abcg8. Animal number for (a–i) and (k,l): Control Sham (n= 5), Control VSG (n= 8), FGF15INT-KOSham (n= 8), FGF15INT-KOVSG (n= 5). Animal number for j: Control Sham (n= 5), Control VSG (n= 8), FGF15INT-KOSham (n= 7), FGF15INT-KOVSG (n= 5). Data are shown as means ± SEM. *p< 0.05 (two-way ANOVA with Tukey’s post hoc test). 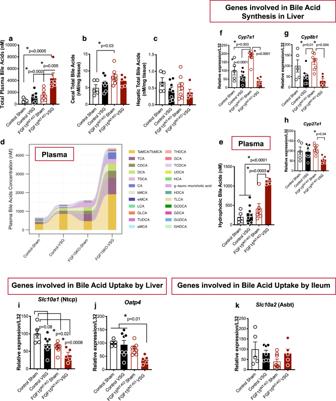Fig. 6: Intestinal FGF15 regulates enterohepatic bile acid metabolism following VSG. aTotal plasma bile acid levels.bCecal contents total bile acid levels.c. Hepatic total bile acids.dPlasma bile acid composition.eHydrophobic plasma bile acid levels. Hepatic RNA expression of bile acid synthesis genes.fCyp7a1,gCyp8b1andhCyp27a1. Hepatic RNA expression of bile acid uptake genesiSlc10a1(coding for Ntcp) andjOatp4.kIleum RNA expression of bile acid uptake geneSlc10a2(coding for Asbt). Animal number for (b), (c), (f–j): Control Sham (n= 5), Control VSG (n= 8), FGF15INT-KOSham (n= 8), FGF15INT-KOVSG (n= 5). Animal number for (a), (d), (e): Control Sham (n= 5), Control VSG (n= 7), FGF15INT-KOSham (n= 6), FGF15INT-KOVSG (n= 5). Animal number for k: Control Sham (n = 5), Control VSG (n= 7), FGF15INT-KOSham (n= 8), FGF15INT-KOVSG (n= 5). Data are shown as means ± SEM. *p< 0.05 (two-way ANOVA with Tukey’s post hoc test). 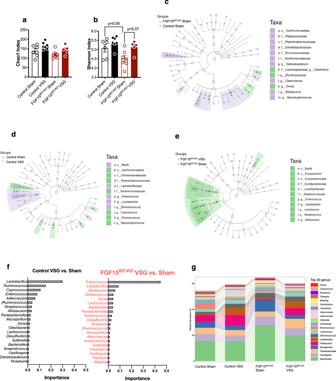Fig. 7: Intestinal FGF15 modulates microbiota in cecal content. aChao1 abundance andbShannon index diversity of the gut microbiota in the cecal contents. LEfSex analysis depicting nodes within the bacterial taxonomic hierarchy that are enriched in cecal microbiota fromcControl Sham versus FGF15INT-KOSham anddControl Sham versus VSG andeFGF15INT-KOSham versus VSG. Diagrams generated by LEfSe indicating differences atphylum,order,class,family, andgenuslevels between the two groups.fTop-ranked taxa atgenuslevel identified by random forest analysis according to their ability to discriminate the microbiota of Sham and VSG mice per genotype in decreasing order of discriminatory importance. A comparison of the abundance of markers in VSG relative to Sham counterparts in each genotype.g. Differences in relative abundance of taxa atgenuslevel. Animal number Control Sham (n= 6), Control VSG (n= 7), FGF15INT-KOSham (n= 7), FGF15INT-KOVSG (n= 5). Data in (a,b) are shown as means ± SEM. *p< 0.05 (two-way ANOVA with Tukey’s post hoc test). 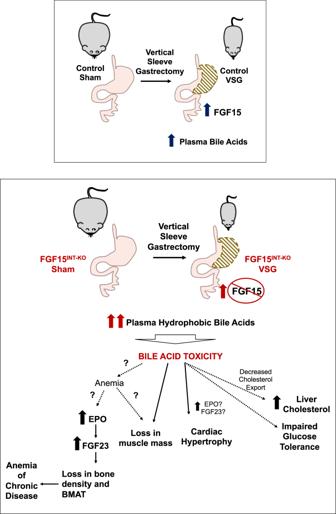Fig. 8: Intestinal-derived FGF15 protects against deleterious effects following sleeve gastrectomy in mice. VSG leads to an increase in ileal expression ofFGF15and total plasma bile acids. In the absence of intestinally derived FGF15 (FGF15INT-KO), VSG leads to an even greater increase in circulating total and specifically, hydrophobic bile acids. We speculate that the increase in hydrophobic bile acids leads to bone marrow dysfunction, which increases EPO and FGF23 levels that likely contribute to potentially serious loss of bone mass, bone marrow adipose tissue (BMAT), inducing anemia of chronic disease. FGF15INT-KOVSG mice have a loss of muscle mass and cardiac hypertrophy, as a result of bile acid toxicity or secondary to anemia of chronic disease. FGF15INT-KOVSG mice also have increased hepatic cholesterol and they do not show improved glucose tolerance following VSG. Reporting summary Further information on research design is available in the Nature Research Reporting Summary linked to this article.